Molecular origin of high field-effect mobility in an indacenodithiophene–benzothiadiazole copolymer One of the most inspiring and puzzling developments in the organic electronics community in the last few years has been the emergence of solution-processable semiconducting polymers that lack significant long-range order but outperform the best, high-mobility, ordered semiconducting polymers to date. Here we provide new insights into the charge-transport mechanism in semiconducting polymers and offer new molecular design guidelines by examining a state-of-the-art indacenodithiophene–benzothiadiazole copolymer having field-effect mobility of up to 3.6 cm 2 V −1 s −1 with a combination of diffraction and polarizing spectroscopic techniques. Our results reveal that its conjugated planes exhibit a common, comprehensive orientation in both the non-crystalline regions and the ordered crystallites, which is likely to originate from its superior backbone rigidity. We argue that charge transport in high-mobility semiconducting polymers is quasi one-dimensional, that is, predominantly occurring along the backbone, and requires only occasional intermolecular hopping through short π-stacking bridges. Organic field-effect transistors (OFETs) based on solution-processable semiconducting polymers [1] , [2] , [3] , [4] , [5] are emerging as a promising candidate for next-generation electronics applications such as flexible display backplanes [6] , [7] and logic circuits [8] , [9] , [10] . Within the past decade, significant efforts in material design have boosted the OFET mobility ( μ ) achievable from semiconducting polymers by more than an order of magnitude, from μ ≤0.1 cm 2 V −1 s −1 exhibited by regioregular poly(3-hexylthiophene) (P3HT) [11] to μ ≥1 cm 2 V −1 s −1 by a number of polymers [12] , [13] , [14] , [15] , [16] , [17] , [18] . More interestingly, in recent years there has been a dramatic change in the semiconductor design motifs employed to optimize carrier mobilities. In analogy with models for small-molecule-based OFETs, such as those made from pentacene [19] , [20] , it has long been believed that outstanding device performance originates from highly ordered structures with optimally oriented domains. Early semiconducting polymers such as regioregular P3HT [11] , poly(3,3′-dialkyl-quaterthiophene) [21] and poly(2,5-bis(thiophen-2-yl)thieno[3,2-b]thiophene) (pBTTT) [22] were thus designed to achieve significant long-range order. Specifically, a two-dimensional (2D) in-plane packing motif [11] , [23] composed of lamellae of edge-on, π-stacked conjugated backbones spaced by lamellae of alkyl side chains stacking along the substrate normal was thought to be critical to achieving high mobility, because the two active charge-transport pathways, that is, those along the conjugated backbone and π-stacking directions, are both aligned parallel to the transistor channel area. This motif renders pBTTT a benchmark mobility of μ ≈1 cm 2 V −1 s −1 (ref. 12 ) but has hardly led to further advances. In contrast, more recent semiconducting polymers with alternating donor–acceptor backbone structures appear to have a less pronounced or even an undetectable long-range order, yet exhibit mobilities significantly >1 cm 2 V −1 s −1 (refs 15 , 16 , 17 ). Representative materials in this category include copolymers incorporating thienothiophene–diketopyrrolopyrrole ( μ max ≈2 cm 2 V −1 s −1 ) (ref. 15 ), bithiophene–isoindigo ( μ max ≈2.5 cm 2 V −1 s −1 ) (ref. 16 ) or cyclopentadithiophene–benzothiadiazole ( μ max ≈3.3 cm 2 V −1 s −1 ) (ref. 17 ) moieties. Moreover, accumulating evidence that challenges the superiority of the 2D in-plane packing motif has emerged when two films with same or similar chemical structures but disparate molecular packing behaviour are compared [16] , [24] , [25] , [26] . These intriguing findings signify a lack of comprehension of what is essential to achieving high mobility besides long-range order. To facilitate future efforts in material development towards rational molecular design, new insights into the charge-transport mechanism in high-mobility semiconducting polymers are highly demanded. Described by McCulloch and coworkers [13] , [14] , an indacenodithiophene–benzothiadiazole (C 16 IDT-BT) copolymer exhibited μ ≈1 cm 2 V −1 s −1 and an X-ray diffraction pattern consisting of weak and broad peaks that likely stem from highly defective lamellar- and π-stacking, which classifies C 16 IDT-BT as being among the before-mentioned high-mobility but apparently substantially disordered donor–acceptor copolymers. In this work, we report significant progress in improving the OFET mobility of C 16 IDT-BT to an extraordinarily high level (up to ≈3.6 cm 2 V −1 s −1 ) by increasing its molecular mass, and demonstrate its applicability in constructing unipolar logic circuits. To uncover the structure–property relationships for C 16 IDT-BT and therefore shed light on charge-transport mechanism in recent high-mobility semiconducting polymers in general, we perform a detailed study of the orientational order of the entire film using polarizing spectroscopies. Quantitative comparison with the 2D diffraction of the ordered regions reveals a consistency of π-conjugated plane orientation between the crystalline and non-crystalline regions, indicating a comprehensive local molecular order. This finding leads to the hypothesis that quasi-1D transport along the backbone, with intermittent π linkages to adjacent chains, is sufficient for high mobility. Electrical performance Top-gate, bottom-contact (TGBC) OFET devices (Fig. 2a) using C 16 IDT-BT (shown in Fig. 1 ) as the active material gave OFET characteristics ( Fig. 2b ) that were an almost ideal fit to the gate voltage (or carrier density)-independent model [27] , in contrast to some other recently reported polymer OFETs that exhibited significant deviations from the ideal transistor equations [28] . Therefore, μ can be unambiguously estimated by taking first and second derivatives of the drain current for linear and saturation regimes ( Fig. 2c ), respectively, giving room-temperature mobilities of 1.5±0.2 cm 2 V −1 s −1 (linear) and 2.0±0.2 cm 2 V −1 s −1 (saturation) with ON/OFF ratios of up to 10 6 from 10 devices with variable channel lengths L =30–100 μm and a constant channel width W =1 mm fabricated at Imperial College London. The maximum mobilities were measured to be 2.0 cm 2 V −1 s −1 (linear) and 3.6 cm 2 V −1 s −1 (saturation) in a device with L =20 μm. Moreover, the device performance of C 16 IDT-BT exhibited the cross-lab reproducibility necessary for electronics applications, because similar saturation mobilities of 2.2±0.2 cm 2 V −1 s −1 were obtained from a second set of four TGBC devices ( L =20 μm and W =1 mm) independently fabricated and tested at the University of Cambridge. These materials support more complex electronic devices as well ( Supplementary Fig. S1 ). We note that the enhancement in mobility by two- to threefolds with respect to our earlier reports [13] , [14] might be attributed to the increased molecular mass [17] , [29] and smaller polydispersity (PDI). Hence, further mobility enhancement can be anticipated from fractionated materials with higher molecular masses and narrower PDIs, as supported by mobilities beyond 5 cm 2 V −1 s −1 obtained from our preliminary electrical characterization of C 2 C 6 IDT-BT, which has the same backbone structure with shorter, branched alkyl side chains. 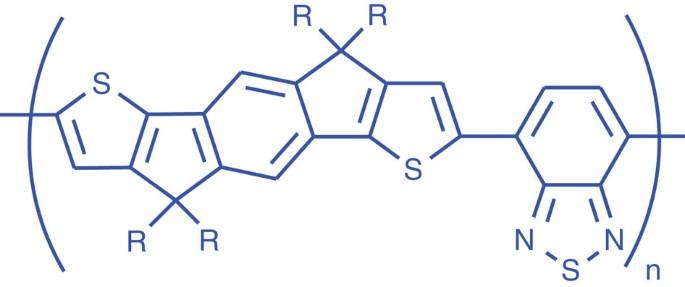Figure 1: Molecular structure of C16IDT-BT. R=Hexadecyl. Figure 1: Molecular structure of C 16 IDT-BT. R=Hexadecyl. 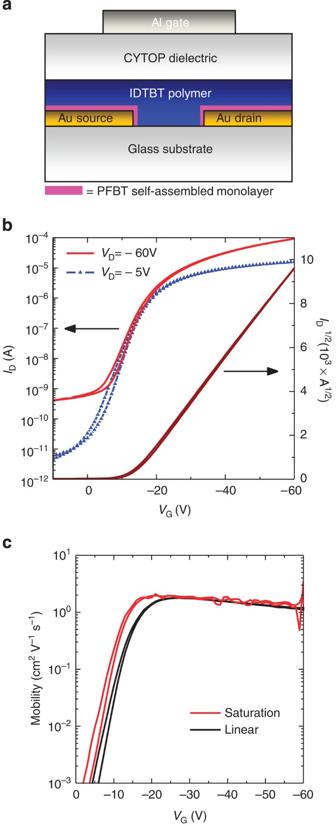Figure 2: Room-temperature OFET characteristics for C16IDT-BT. (a) TGBC device configuration, (b) transfer curves and (c) mobility calculation based on first derivative of the linear regime transfer curve and second derivative of the saturation regime transfer curve. The dimensions of the device areL=50 μm andW=1 mm. Full size image Figure 2: Room-temperature OFET characteristics for C 16 IDT-BT. ( a ) TGBC device configuration, ( b ) transfer curves and ( c ) mobility calculation based on first derivative of the linear regime transfer curve and second derivative of the saturation regime transfer curve. The dimensions of the device are L =50 μm and W =1 mm. Full size image The second set of devices were also subjected to measurements in the temperature range between 200 and 300 K, showing thermally activated charge transport ( Fig. 3 ); that is, lowering the temperature led to reduced currents while the transistors still exhibited a high ON/OFF ratio and saturation behaviour. The saturation mobilities at different temperatures were extracted as described above and are shown in an Arrhenius plot ( Fig. 3c ), which allowed the extraction of an activation energy of 61 meV. The activation energy might be somewhat enlarged partly by disorder in the polymer film. Nevertheless, its value is fairly close to those obtained from high-molecular-mass pBTTT [30] and regioregular P3HT [29] devices, implying that the charge transport in C 16 IDT-BT might be limited by similar processes such as interchain hopping that govern their activation energies, in spite of the apparently different morphology exhibited by C 16 IDT-BT [13] as compared with pBTTT [23] and P3HT [11] , [29] . 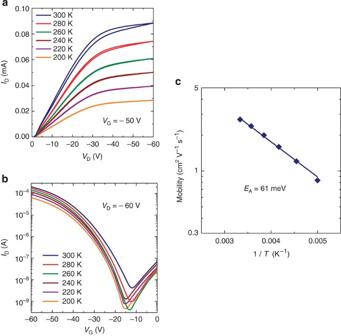Figure 3: OFET characteristics for C16IDT-BT. (a) Output curves with temperature dependence. (b) Transfer curves with temperature dependence. (c) An Arrhenius plot. The dimensions of the device areL=20 μm andW=1 mm. Uncertainty for temperature measurement is ±1%. Figure 3: OFET characteristics for C 16 IDT-BT. ( a ) Output curves with temperature dependence. ( b ) Transfer curves with temperature dependence. ( c ) An Arrhenius plot. The dimensions of the device are L =20 μm and W =1 mm. Uncertainty for temperature measurement is ±1%. Full size image Polarizing spectroscopies C 16 IDT-BT films exhibit only weak and broad low-order lamellar and π-stacking peaks and no detectable thermal transitions in preliminary differential scanning calorimetric results [13] . For such non-crystalline films, polarizing spectrocopies that average both crystalline and non-crystalline regions, such as variable-angle spectroscopic ellipsometry (VASE) and near-edge X-ray absorption fine structure (NEXAFS) spectroscopy, are necessary to obtain a complete picture of the microstructure. For films that are isotropic in-plane, these techniques provide quantitative insight into the second moment of the orientation distribution with respect to surface normal, θ , of the relevant transition dipole ( cos 2 θ ). VASE measurements were recorded to provide information about the orientation of the π–π* transition dipole vector [31] , [32] , [33] —namely, the backbone orientation in the case of linear polymers. In a typical VASE experiment, both the amplitude ratio (Ψ) and phase shift (Δ) for light polarized parallel or perpendicular to the plane of incidence are recorded as a function of wavelength at multiple incidence angles. Dielectric function (or complex refractive index) and film thickness can be extracted from the model that best fits the Ψ and Δ data. Similar to many other spin-cast semiconducting polymers, C 16 IDT-BT is best described by a uniaxial model [23] , [31] , [32] , [33] , [34] , [35] exhibiting no preferred in-plane backbone orientation and different dielectric functions for the in-plane ( ε x−y ) and out-of-plane ( ε zz ) directions. 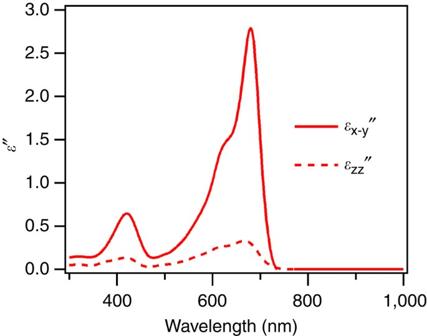Figure 4: VASE measurements of an C16IDT-BT film. The imaginary part of the dielectric function based on a uniaxial model. Figure 4 shows the corresponding imaginary (absorptive) part of the modelled dielectric function. The resemblance in line shape between ε ′′ x−y and ε ′′ zz suggests that the microstructure responsible for the transitions is similar. [33] In such a case, the dichroic ratio ε ′′ zz / ε ′′ x−y can be used to quantify the average backbone orientation relative to the substrate normal ( θ bb ) from a simple calculation [33] : ε ′′ zz / ε ′′ x−y =2 × cos 2 θ bb / sin 2 θ bb . By integrating the area over the wavelength range between 466 and 720 nm, ε ′′ zz / ε ′′ x−y =0.17 is obtained, indicating cos 2 θ bb =0.078. The second moment does not uniquely define the orientation distribution. It may, however, be pictured using simplified models such as a uniform distribution of angles between 61° and 90° or a bimodal system that is 92% completely in-plane with an 8% tail-on minority component. Note that C 16 IDT-BT is not among the most anisotropic semiconducting polymers; pBTTT [23] and DPPT-TT [25] , a diketopyrrolopyrrole–thienothiophene copolymer, both exhibited ε ′′ zz / ε ′′ x−y ≤0.05. C 16 IDT-BT does, however, show substantial backbone alignment parallel to the substrate plane. Figure 4: VASE measurements of an C16IDT-BT film. The imaginary part of the dielectric function based on a uniaxial model. Full size image NEXAFS spectroscopy [36] was performed to analyse the average orientation of the conjugated plane of C 16 IDT-BT by measuring the 1s-π* resonance intensity as a function of incidence angle ( Θ i ) of the linearly polarized soft X-ray beam [23] , [33] . In its partial electron yield data collection mode, NEXAFS only probes the topmost few nanometres of the films analysed, which essentially constitute the charge-transport channel in a top-gate OFET device. The same measurements can also be recorded using films delaminated by sheets of polydimethylsiloxane elastomer to characterize the average orientation of the conjugated plane at the buried interface [33] . In materials in which the interface orientation may be distinct from the bulk, transmission NEXAFS can also be used [37] ; near-surface depth profiling of orientation with NEXAFS, however, gave us no reason to believe that C 16 IDT-BT has a distinct interface orientation. 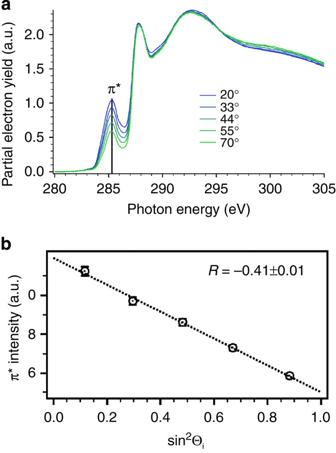Figure 5: Carbon K-edge NEXAFS spectra of C16IDT-BT. (a) NEXAFS spectra recorded at five incidence angles (Θi) for the top surface of C16IDT-BT films. (b) The π* intensity as a function of sin2Θiis well fitted into a straight line. NEXAFS partial electron yield and photon energy have standard uncertainties of ±2% and ±0.1 eV, respectively. Figure 5 shows NEXAFS spectra acquired from the top interface of a C 16 IDT-BT film cast on Si, which is the interface relevant to the above-mentioned device performance. The π* intensity is found to be strongly dependent on Θ i ; that is, it decreases significantly as Θ i increases, a trend that is opposite to what has been reported for most high-mobility semiconducting polymers [23] , [25] , [32] . This trend signifies preferentially face-on orientation of the conjugated plane. Quantification of the dichroism induced by such conjugated plane orientation is usually expressed by a dichroic ratio R , defined by the difference between the extrapolated intensities at 90° and 0° incidence normalized by their sum. R typically varies from 0.7 (extremely edge-on) to −1.0 (perfectly face-on), with R =0 corresponding to isotropic distribution or an orientation of all conjugated planes at precisely the magic angle (54.7°). R =–0.41 was calculated for the top surface of C 16 IDT-BT. The buried interface of C 16 IDT-BT showed similar angular dependence of the π* intensity and an even stronger preference for face-on orientation of the conjugated planes ( R =–0.56). To our knowledge, these values mark C 16 IDT-BT as the most face-on semiconducting polymer reported so far. As a point of comparison, R for C 16 IDT-BT is almost identical to those obtained from chemically derived graphene films ( R ranges from −0.47 to −0.59) [38] . If we take R =−0.41 and −0.56 as the upper and lower limits for the dichroic ratio of the film, respectively, the moment of the angle that the 1s-π* transition dipole is tilted away from the substrate normal ( cos 2 θ π ) can be calculated as being between ≈0.57 and ≈0.67 (ref. 23 ). Similar to the average backbone tilt extracted from VASE, these numbers do not define a specific orientation distribution of the conjugated plane, but may be interpreted, for instance, as a uniform distribution of angles between 0° and ≈56° or a bimodal system that has ≈60% of the π-planes face-on and the rest edge-on. Figure 5: Carbon K-edge NEXAFS spectra of C 16 IDT-BT. ( a ) NEXAFS spectra recorded at five incidence angles ( Θ i ) for the top surface of C 16 IDT-BT films. ( b ) The π* intensity as a function of sin 2 Θ i is well fitted into a straight line. NEXAFS partial electron yield and photon energy have standard uncertainties of ±2% and ±0.1 eV, respectively. Full size image Grazing-incidence X-ray diffraction Although polarizing spectroscopies provide insight into the average orientational order, they do not provide significant details on molecular distances. This can be extracted from unit cell sizes in crystalline regions. The 2D diffraction image acquired from C 16 IDT-BT ( Fig. 6a ) resembles our earlier results from materials with the same chemical structure but a lower molecular mass [13] . C 16 IDT-BT diffracts very weakly compared with pBTTT [39] or P3HT [11] , [29] . Coexistence of face-on and edge-on crystalline domains can be inferred from the appearance of both the (200) ( q ≈0.48 Å −1 ) and (010) ( q ≈1.65 Å −1 ) reflections in the out-of-plane direction, corresponding to d -spacing values of 2.6 and 0.38 nm for lamellar stacking of the backbones along the alkyl side chain direction and π-stacking, respectively. The assignment of the (200) reflection is corroborated by grazing-incidence X-ray diffraction (GIXD) patterns obtained from IDT-BT polymers grafted with shorter alkyl side chains ( Supplementary Fig. S2 ), because the spacing scales with the side chain length (that is, hexadecyl>octyl>ethylhexyl>methylbutyl). Both the (200) and (010) reflections appear as broad and wide arcs, suggesting that the corresponding crystallites are small and have a large orientation distribution. This contrasts significantly with the highly oriented and ordered microstructure exhibited by pBTTT and similar early-generation semiconducting polymers [23] . The estimated correlation lengths based on Scherrer’s equation gave 4.9 nm (or only ≈2 lamellae) and 3.3 nm (or 8–9 π-stacks) for the (200) and (010) reflections, respectively. Note that these correlation lengths do not equate to crystallite dimensions, because other factors such as non-uniform crystal strain and paracrystallinity can also contribute to peak broadening, but they do indicate substantial disorder in the out-of-plane direction. The π-stacking repeat distance is comparable to that exhibited in most highly crystalline, well-ordered polymers [39] , indicating that the disordered side chains do not inhibit local π-stacking, consistent with the larger, in terms of repeat units, (010) correlation length. 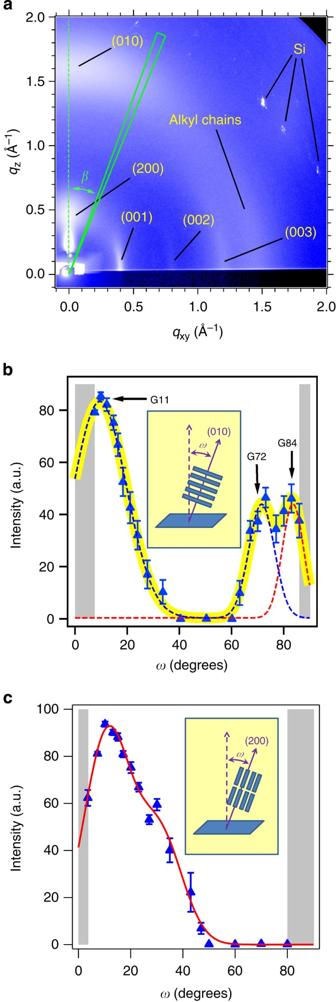Figure 6: GIXD from C16IDT-BT. (a) 2D detector image. (b,c) Sinω-corrected pole figures for the (010) and (200) reflections, respectively. Data inbare fitted by three Gaussian peaks (marked as G11, G72 and G84), with the thick yellow trace showing the overall fitting and the two dashed traces showing a possible deconvolution of the intensities from the (010) (blue) and (004) (red) reflections. Data incare fitted by two overlapping Gaussian peaks. The error bars inbandcdenote the s.d. from the coefficients extracted from multiple-Lorentzian peak fitting of the wedge cuts. The insets inbandcillustrate howωis defined in each pole figure. The grey-shaded areas inbandcdenote the ranges ofωthat are either inaccessible from GIXD measurements (low angles) or where the field-enhancement effect along the horizon of the image detector dominates (high angles). Figure 6: GIXD from C 16 IDT-BT. ( a ) 2D detector image. ( b , c ) Sin ω- corrected pole figures for the (010) and (200) reflections, respectively. Data in b are fitted by three Gaussian peaks (marked as G11, G72 and G84), with the thick yellow trace showing the overall fitting and the two dashed traces showing a possible deconvolution of the intensities from the (010) (blue) and (004) (red) reflections. Data in c are fitted by two overlapping Gaussian peaks. The error bars in b and c denote the s.d. from the coefficients extracted from multiple-Lorentzian peak fitting of the wedge cuts. The insets in b and c illustrate how ω is defined in each pole figure. The grey-shaded areas in b and c denote the ranges of ω that are either inaccessible from GIXD measurements (low angles) or where the field-enhancement effect along the horizon of the image detector dominates (high angles). Full size image In stark contrast to the diffuse out-of-plane peaks, the majority of in-plane diffracted intensity is observed as a series of rod-like peaks at q ≈0.4, 0.8 and 1.2 Å −1 , corresponding to d -spacing ≈1.57 nm and consistent with diffraction along the backbone, (00 l ), based on the repeat unit length calculated by force field calculations (1.61 nm). Again, the assignment of these backbone peaks can be corroborated by GIXD patterns obtained from other IDT-BT polymers with shorter side chains ( Supplementary Fig. S2 ), as the peak positions are identical for the entire side chain series. The shape of these peaks is indicative of highly oriented backbones that are parallel to the substrate plane, which has also been observed in pBTTT [39] and P(NDI2OD-T2) (refs 40 , 41 ), a high-mobility electron-transporting polymer. The correlation length estimated from full-width at half-maximum of the (001) peak is 22 nm or ≈14 repeat units, implying significant ordering along the backbone direction possibly induced by coplanarity of the conjugated rings. There are no clearly discernible in-plane (h00) reflections as one would expect from face-on crystallites, possibly because of the following fact: for a given azimuthal tilt, the fraction of crystals probed in GIXD experiments decreases as the azimuthal tilt increases. Hence, the number of crystallites giving rise to in-plane reflections is substantially undercounted [42] , [43] . To quantify the orientation distribution of C 16 IDT-BT crystallites, we constructed a pole figure for the (010) reflection, as shown in Fig. 6b . Details are provided in Supplementary Note 1 and Supplementary Fig. S3 . Briefly, wedge cuts were first taken at a series of detector angles, β (illustrated in Fig. 6a ). The (010) intensities were then extracted by a curve-fitting procedure [43] to separate the scattering intensities that overlap with the peak of interest. The deconvoluted intensities, after appropriate corrections, were plotted against azimuthal angle ω , which is the angle between a crystallite’s π-stacking direction and the substrate normal, illustrated in Fig. 6b . The corrections include a minor polarization correction [44] and the geometric sin ω correction [43] , whereas the absorption correction is considered negligible. It is worth noting that ω does not equal β at small values as a result of fixed incidence beam and the curved surface of the Ewald sphere [43] , [44] ; for example, β =0° corresponds to the Bragg angle (for q =1.65 Å −1 , ω ≈7°). This means that the crystallites with ω less than the Bragg angle cannot be detected by 2D GIXD. A local specular experiment can complement GIXD by providing intensities for the crystallites with ω less than the Bragg angle [44] , [45] , [46] . However, the signal-to-noise ratio was found unsatisfactory in such an experiment for the (010) reflection. Therefore, the region for ω <≈7° was marked as a grey-shaded area in Fig. 6b . We note that intensities for ω near 90° also cannot be properly acquired, because of field-enhancement effect along the horizon of the image detector and shadowing from the sample, leading to a second grey-shaded area in Fig. 6b . In spite of the presence of these two inaccessible regions, we can safely assume that the intensities at ω =0° and 90° can be extrapolated [43] , because the lack of strong intensities in local specular experiments suggests that highly oriented crystallites are unlikely to occur in C 16 IDT-BT. As shown in Fig. 6b , the orientation distribution of intensities at q =1.65 Å −1 is well fitted by three Gaussians centred at ω ≈11°, 72° and 84° (denoted in Fig. 7b and the following text as G11, G72 and G84). Although G11 can be attributed to the (010) reflection of the nominally face-on crystallites unambiguously, G72 and G84 might not completely originate from the (010) reflection of the edge-on crystallites. This complication arises from the possibility that there might be an in-plane (004) reflection at almost identical position ( q ≈1.6 Å −1 ), and the overall weak intensities for ω >60° make it extremely difficult to distinguish between contributions related to the (010) and (004) reflections in this ω range. To deduce the in-plane (010) intensities, we constructed a pole figure for the (200) reflection ( Fig. 6c ). As the same edge-on crystallites are expected to exhibit (h00) and (010) reflections with similar orientation distribution breadth at nominally orthogonal angles, the second moment of orientation distribution of in-plane (010) intensities ( cos 2 ω 010ip ) can be calculated from that of (200) intensities ( cos 2 ω 200 ) as follows: cos 2 ω 010ip = cos 2 ( ω 200 +90°) = sin 2 ω 200 ) =1– cos 2 ω 200 ) =1–0.86=0.14. This value is quite close to the calculated second moment of orientation distribution based solely on G72 (0.13). It is thus tempting to assume that G11 and G72 represent the pole figure for the (010) reflection, and G84 is related to the (004) reflection. Such assignments agree with the expectation that (00l) reflections should appear near ω ≈90°, but are inconsistent with the much narrower breadth of G72 (≈20°) as compared with the orientation distribution of the (200) reflection (≈40°). On the other hand, the combined breadth of G72 and G84 (>30°) is comparable to the orientation distribution of the (200) reflection, but the calculation of the second moment of orientation distribution taking both G72 and G84 into account (0.08) generates a non-negligible deviation from cos 2 ω 010ip . These calculations suggest that the (010) and (004) intensities may be convoluted in a more complicated way. Nevertheless, both the thick yellow trace and the dashed blue trace in Fig. 6b can be regarded as approximations to the actual pole figure of the (010) reflection. For these two circumstances, cos 2 ω 010 was calculated to be 0.63 (yellow trace) and 0.74 (blue trace), corresponding to ω 010 values of ≈38° and ≈31°, respectively (or a preferential face-on orientation of the conjugated ring planes). 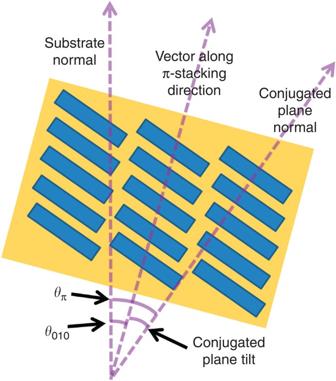Figure 7: Illustration of the unequivalence ofθ010andθπ. Schematic of a crystallite viewed along the backbone axis. Figure 7: Illustration of the unequivalence of θ 010 and θ π . Schematic of a crystallite viewed along the backbone axis. Full size image It is possible to deduce backbone rigidity by comparing orientation measurements from NEXAFS and GIXD. With the figures of merit θ 010 and θ π obtained from NEXAFS and GIXD measurements, respectively, we can compare the orientation of the conjugated planes between crystallites and the volume average of both crystalline and non-crystalline fractions. It is noteworthy that θ 010 is not necessarily equivalent to θ π (illustrated in Fig. 7 ), as conjugated plane tilting within the unit cell was found common and energetically favourable for semiconducting polymers [23] , [47] , [48] . In the cases of PBTTT, poly(3,3′-dialkyl-quaterthiophene) and P3HT, the optimum tilting angle between the conjugated plane normal and the (010) crystal direction was determined to be between 20° and 30° (refs 23 , 47 ). To account for such tilting, we calculated a series of θ π GIXD values by considering different tilting angles for the approximation of the (010) pole figure, assuming that G84 comes from the (004) reflection, as shown in Fig. 8a . As this approximation shows bimodal orientation distributions, the corresponding θ π GIXD only exhibits moderate dependence on conjugated plane tilting. θ π extracted from NEXAFS measurements is not readily usable for comparison, because backbones are on average tilted 16° away from the substrate plane (VASE measurements), whereas the backbones within crystallites are strictly parallel to it. To make a sensible comparison, the contribution to θ π NEXAFS by this backbone tilting was excluded by an approach described in Supplementary Fig. S4 , leading to a corrected θ π NEXAFS range from ≈38 to ≈32 as highlighted by the pink area in Fig. 8a . 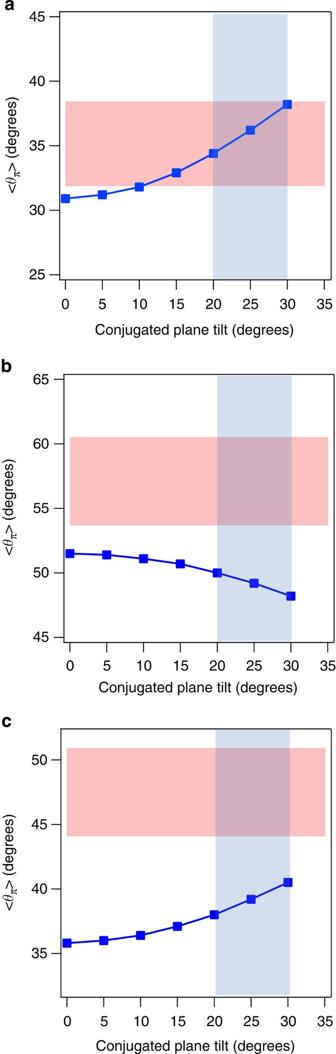Figure 8: Comparison of orientation from GIXD and NEXAFS. The average orientation of the conjugated plane calculated from GIXD (θπGIXD) as a function of the angle between the (010) reflection and the conjugated plane normal for (a) C16IDT-BT, (b) fast-dried, non-annealed P3HT and (c) fast-dried, non-annealed DPPT-T. The solid lines are guides to the eye. The upper and lower bounds of the pink areas inadenote the average orientation of the conjugated plane based on the corrected NEXAFS spectra (θπNEXAFS) of top and buried interfaces, respectively. The pink areas inbandcare artificially broadened in the vertical direction to match that ofa, because P3HT and DPPT-T exhibit smaller differences between top and buried interfaces in NEXAFS. The light blue areas highlight the conjugated plane tilt range between 20° and 30°, that is, the most probable conjugated plane tilt range for alkylated polythiophenes. Figure 8: Comparison of orientation from GIXD and NEXAFS. The average orientation of the conjugated plane calculated from GIXD ( θ π GIXD ) as a function of the angle between the (010) reflection and the conjugated plane normal for ( a ) C 16 IDT-BT, ( b ) fast-dried, non-annealed P3HT and ( c ) fast-dried, non-annealed DPPT-T. The solid lines are guides to the eye. The upper and lower bounds of the pink areas in a denote the average orientation of the conjugated plane based on the corrected NEXAFS spectra ( θ π NEXAFS ) of top and buried interfaces, respectively. The pink areas in b and c are artificially broadened in the vertical direction to match that of a , because P3HT and DPPT-T exhibit smaller differences between top and buried interfaces in NEXAFS. The light blue areas highlight the conjugated plane tilt range between 20° and 30°, that is, the most probable conjugated plane tilt range for alkylated polythiophenes. Full size image Interestingly, the blue trace derived from our tentative in-plane (010) peak assignment falls almost entirely within the highlighted region, especially for the conjugated plane tilt range between 20° and 30° ( Fig. 8a ). The same analysis based on the assumption that the (004) reflection is completely absent also leads to partial overlap and small discrepancy between the calculated trace and the highlighted region ( Supplementary Fig. S5 ). This agreement between θ π NEXAFS and θ π GIXD suggests that the conjugated planes in C 16 IDT-BT are oriented in similar ways irrespective of whether their environments are crystalline or non-crystalline. Such resemblance can be expected from intrinsically rigid chains, because they do not require crystallization to preserve conjugated ring coplanarity. The superior backbone rigidity of C 16 IDT-BT can also be inferred from the following facts: (1) the line shape of ε′′ x−y and ε′′ zz obtained from VASE measurements ( Fig. 4 ) is very similar, suggesting that the chains responsible for out-of-plane absorption, which are likely to be non-crystalline, are as rigid as those parallel to the substrate plane, which are likely to be at least partially crystalline; (2) the change in the ultraviolet-visible absorption spectrum from solution to thin film is unremarkable [13] , which might imply that rigid chains, either individual or aggregated, are carried over from solution to thin film; and (3) the small torsional angle (≈7) between conjugated rings has been predicted from density functional theory calculations [49] . Although rigid chains such as C 16 IDT-BT tend to exhibit orientation consistency ( Fig. 8a ), more twistable chains are likely to have disparate θ π NEXAFS and θ π GIXD , because the backbones are rigidified only in the crystallites and subject to torsional disorder in non-crystalline regions. This can be demonstrated by the absence of overlap between the blue traces ( θ π GIXD ) and the highlighted areas ( θ π NEXAFS ) in Fig. 8b,c , where fast-dried, non-annealed films of P3HT [24] and DPPT-T, a DPP-terthiophene copolymer [25] , are analysed. This quantitative comparison of NEXAFS and GIXD results can therefore be applied as a method to reveal backbone rigidity in a variety of semiconducting polymers. C 16 IDT-BT exhibits field-effect mobilities more than an order of magnitude higher compared with those obtained from as-processed P3HT [24] and DPPT-T [25] , which cannot be correlated with crystallinity or the π-stacking crystal order. We argue that, in the absence of significant long-range order, backbone rigidity stands out as the best candidate to account for superior OFET mobilities measured in C 16 IDT-BT. In other words, because the backbones have a leading role in constituting the charge-transport pathway, only occasional π-stacking is required to relay the charge carriers. As the orientation distribution is comprehensive between crystalline and non-crystalline regions, we can surmise that the local molecular order is similar, implying tight (0.38 nm separation) π-coupling even in the non-crystalline regions. This quasi-1D charge-transport model may well apply to the whole class of high-mobility semiconducting polymers that appear substantially disordered. In materials such as pBTTT and P3HT, it seems probable that the π-stacking necessary for charge transport between chains would occur more often within the well-ordered domains that are typically observed. In C 16 IDT-BT, ‘crystalline’ regions of commonly well-ordered backbones are not observed, but perhaps may occur at very small length scales. Regardless, interchain charge hopping is demonstrably sufficient for facile charge transport. Considering the high degree of paracrystallinity along the π-stacking direction in pBTTT revealed by advanced X-ray line shape analysis [50] and the charge-transport anisotropy observed in oriented pBTTT films [51] , we might conjecture that the primary effect of the lamellar packing motif in pBTTT and other early-generation materials enhances the coplanarity of the backbones (pBTTT backbone peaks have also been observed in GIXD [39] ) instead of promoting a 2D charge-transport network. Regardless of its origin, greater backbone copolanarity would generally promote more intramolecular charge delocalization. This is also consistent with recent reports of good mobility in P3HT films with significant face-on populations [24] . Therefore, the high charge mobilities of C16IDT-BT and pBTTT may both have their origin in backbone copolanarity, differing only in the way this coplanarization is realised. Polymer synthesis C 16 IDT-BT was synthesized via a Suzuki cross-coupling condensation as described earlier [13] , [14] . By performing the polymerization on a larger scale, it is possible to minimize errors in weighing, allowing an exact stoichiometric ratio of monomers. As a result, the polymer was obtained at a high molecular mass of M n ≈80 kg mol −1 , M w ≈160 kg mol −1 , with a PDI of 2, as determined by gel permeation chromatography using narrow PDI polystyrene standards. Device fabrication and thin-film processing TGBC devices were fabricated and tested at both Imperial College London and the University of Cambridge. Thin films (≈20 nm) of C 16 IDT-BT were spin-cast from either chlorobenzene (CB) solutions (5 mg ml −1 ) or 1,2-dichlorobenzene solutions (10 mg ml −1 ) on glass substrates with lithographically patterned and pentafluorobenzenethiol-treated Au source/drain electrodes before a thermal annealing at 150 °C for 10 min for films cast from CB solution or at 200 °C overnight for films cast from 1,2-dichlorobenzene solution. CYTOP (CTL-809M; Asahi Glass) was spin-cast on top of C 16 IDT-BT to yield a dielectric layer (450–800 nm thick). Finally, Au or Al gate electrodes were thermally evaporated on top of CYTOP to complete device fabrication. Because the OFET mobility of C 16 IDT-BT was insensitive to processing parameters, only thin films spin-cast from CB solutions (5 mg ml −1 ) and annealed at 150 °C for 10 min were subjected to diffraction and spectroscopic measurements. For GIXD and NEXAFS, all samples were made on Si 100 wafers with native oxide. For VASE, duplicate films cast on a pair of substrates, namely, Si with native oxide (≈1.7 nm thick) and thermally grown oxide (≈200 nm thick), were both measured to reduce correlations in the extracted dielectric functions. Diffraction and spectroscopic measurements GIXD measurements were performed at the Stanford Synchrotron Radiation Laboratory on beamline 11-3 with an incident energy of 12.7 keV. 2D Diffraction images were collected with an area detector (MAR345 image plate). The samples were housed in a chamber filled with helium during experiments to reduce beam damage and air scattering. Typical exposure times were on the order of ≈10 min. The incidence angle of the X-ray beam was selected to be 0.12°, above the critical angle of the film but below the critical angle of the substrate. NEXAFS spectroscopy was performed at the NIST/Dow soft X-ray material characterization facility, beamline U7A of the National Synchrotron Light Source at Brookhaven National Laboratory. Carbon K-edge spectra were collected in partial electron yield mode with a grid bias of -50 V. Spectra collected at five incidence angles with respect to the surface plane, that is, 20°, 33°, 44°, 55° and 70°, were normalized with respect to carbon concentration by their intensity at 330 eV. VASE was performed at four angles from the surface plane (45°, 35°, 25° and 15°) with an M 2000 series ellipsometer (J.A. Woollam Co., Inc.) housed in a nitrogen glove box and analysed using vendor-supplied software. How to cite this article: Zhang, X. et al. Molecular origin of high field-effect mobility in an indacenodithiophene–benzothiadiazole copolymer. Nat. Commun. 4:2238 doi: 10.1038/ncomms3238 (2013).